Carbon-depleted outer core revealed by sound velocity measurements of liquid iron–carbon alloy The relative abundance of light elements in the Earth’s core has long been controversial. Recently, the presence of carbon in the core has been emphasized, because the density and sound velocities of the inner core may be consistent with solid Fe 7 C 3 . Here we report the longitudinal wave velocity of liquid Fe 84 C 16 up to 70 GPa based on inelastic X-ray scattering measurements. We find the velocity to be substantially slower than that of solid iron and Fe 3 C and to be faster than that of liquid iron. The thermodynamic equation of state for liquid Fe 84 C 16 is also obtained from the velocity data combined with previous density measurements at 1 bar. The longitudinal velocity of the outer core, about 4% faster than that of liquid iron, is consistent with the presence of 4–5 at.% carbon. However, that amount of carbon is too small to account for the outer core density deficit, suggesting that carbon cannot be a predominant light element in the core. Sound velocity and density are important observational constraints on the chemical composition of the Earth’s core. While properties of solid iron alloys have been extensively examined by laboratory studies to core pressures (>136 GPa) [1] , [2] , [3] , little is known for liquid alloys because of experimental difficulties. The core is predominantly molten, and the longitudinal wave (P-wave) velocity of liquid iron alloy is the key to constraining its composition. However, previous static high-pressure and -temperature ( P–T ) measurements of liquid iron alloys were performed only below 10 GPa using large-volume presses [4] , [5] , [6] . Shock wave experiments have been carried out at much higher pressures but only along a specific Hugoniot P–T path [7] , [8] . Carbon is one of the possible light alloying components in the core because of its high cosmic abundance and strong chemical affinity with liquid iron [9] . Its high metal/silicate partition coefficients indicate that thousands of parts per million to several weight percent of carbon could have been incorporated into the core during its formation [9] , [10] , [11] . In addition, recent experimental and theoretical studies [12] , [13] have suggested that solid Fe 7 C 3 may explain the properties of the inner core, in particular its high Poisson's ratio [14] , [15] , supporting the presence of carbon in the core. In this study, we determine the P-wave velocity ( V P ) (equivalent to bulk sound velocity, V Φ , in a liquid) of liquid Fe 84 C 16 at high P–T based on inelastic X-ray scattering (IXS) measurements. Combined with its density data at 1 bar (ref. 16 ) both velocity and density ( ρ ) profiles of liquid Fe 84 C 16 along adiabatic compression are obtained. They are compared with seismological observations, indicating that both V P and ρ in the Earth’s outer core are not explained simultaneously by liquid Fe–C. Longitudinal wave velocity measurements We collected the high-resolution IXS spectra from liquid Fe 84 C 16 (4.0±0.3 wt.% carbon) at static high P–T using both resistance- and laser-heated diamond-anvil cells (Methods; Fig. 1 ). The starting material was synthesized beforehand as a mixture of fine-grained Fe and Fe 3 C at 5 GPa and 1,623 K in a multi-anvil apparatus. Experimental P–T conditions were well above the eutectic temperature in the Fe–Fe 3 C binary system ( Supplementary Fig. 1 ). The carbon concentration in the eutectic liquid is known to be 3.8–4.3 wt.% at 1 bar to 20 GPa (ref. 17 ), almost identical to the composition of our sample. Above 20 GPa, we heated the sample to temperatures comparable or higher than the melting temperature of Fe 3 C, a liquidus phase in the pressure range explored, assuring a fully molten sample. The molten state of the specimen was carefully confirmed, before and after the IXS measurements, by the absence of diffraction peaks from the sample ( Fig. 2 ). We sometimes, depending on a sample volume, were also able to observe the diffuse diffraction signal typical of a liquid. 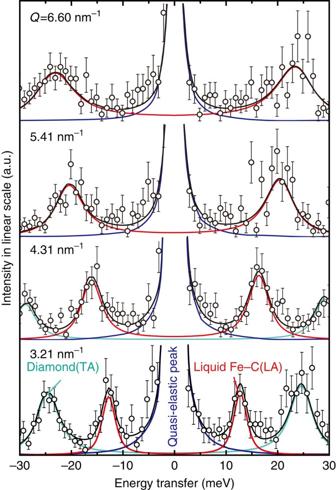Figure 1: Typical inelastic X-ray scattering spectra. These data were collected at 26 GPa and 2,530 K at momentum transfersQ, as indicated. The spectra include three components: a quasi-elastic peak near zero energy transfer (blue), longitudinal acoustic (LA) phonon mode of liquid Fe84C16(red), and transverse acoustic (TA) phonon mode of diamond (turquoise). Figure 1: Typical inelastic X-ray scattering spectra. These data were collected at 26 GPa and 2,530 K at momentum transfers Q , as indicated. The spectra include three components: a quasi-elastic peak near zero energy transfer (blue), longitudinal acoustic (LA) phonon mode of liquid Fe 84 C 16 (red), and transverse acoustic (TA) phonon mode of diamond (turquoise). 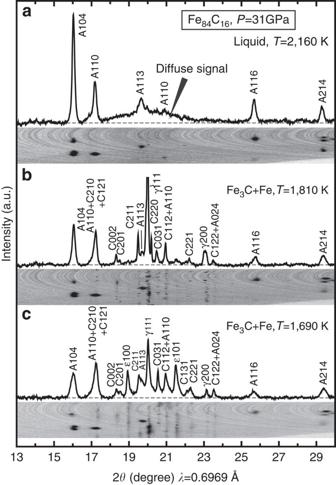Figure 2: X-ray diffraction spectra before and after melting. They were collected at 2,160 K (a), 1,810 K (b) and 1,690 K (c) during heating at 31 GPa. The starting material was composed of Fe (ɛorγ) and Fe3C (c), and the peaks of Al2O3(a) were from a thermal insulator. The coexistence ofɛ- andγ-Fe phases at 1,610 K was due to a sluggish solid–solid phase transition49and the peaks from theɛ-phase were lost at 1,810 K. All sample peaks disappeared between 1,810 and 2,160 K. In addition, the background was enhanced slightly, indicating a diffuse scattering signal from a liquid sample. Full size image Figure 2: X-ray diffraction spectra before and after melting. They were collected at 2,160 K ( a ), 1,810 K ( b ) and 1,690 K ( c ) during heating at 31 GPa. The starting material was composed of Fe ( ɛ or γ ) and Fe 3 C ( c ), and the peaks of Al 2 O 3 ( a ) were from a thermal insulator. The coexistence of ɛ - and γ -Fe phases at 1,610 K was due to a sluggish solid–solid phase transition [49] and the peaks from the ɛ -phase were lost at 1,810 K. All sample peaks disappeared between 1,810 and 2,160 K. In addition, the background was enhanced slightly, indicating a diffuse scattering signal from a liquid sample. Full size image The V P of liquid Fe 84 C 16 was determined between 7.6 and 70 GPa ( Fig. 3 and Supplementary Table 1 ) from dispersion curves for a range of momentum transfer ( Fig. 4 ). It was found to be 15–30% smaller than that of solid Fe (refs 3 , 18 , 19 , 20 ) and Fe 3 C (refs 21 , 22 , 23 ; note that a starting material in the present experiments was a mixture of these solid phases) ( Fig. 5 ), confirming that we measured a liquid sample. The velocities of a fictive solid Fe 84 C 16 alloy are also estimated assuming a linear velocity change between Fe (ref. 24 ) and Fe 3 C (ref. 23 ) indicating that V P drops by 13% upon melting at 2,300 K, a eutectic temperature at 45 GPa (ref. 17 ). Such a velocity change is comparable to that expected for pure Fe. The difference in V Φ between solid and liquid Fe 84 C 16 is very small (1.8%). On the other hand, the V P of our liquid Fe 84 C 16 sample is 3–14% faster at 8–70 GPa than that of liquid Fe determined by shock-wave study [8] ( Fig. 3 ). 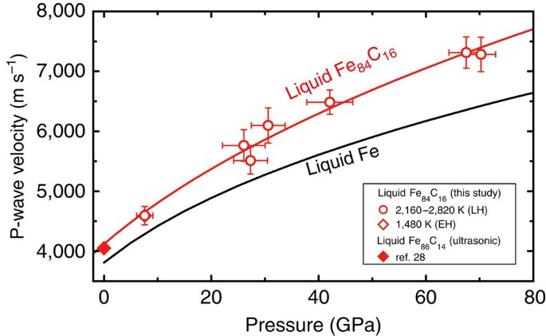Figure 3: Compressional wave velocity of liquid Fe84C16. Open circles, obtained by laser-heated DAC; open diamond, by external-resistance-heated DAC. The data at 1 bar is from ultrasonic measurements28(closed diamond). The red curve represents a thermodynamical fitting result for liquid Fe84C16, compared with the velocity of liquid Fe (black curve)8. Figure 3: Compressional wave velocity of liquid Fe 84 C 16 . Open circles, obtained by laser-heated DAC; open diamond, by external-resistance-heated DAC. The data at 1 bar is from ultrasonic measurements [28] (closed diamond). The red curve represents a thermodynamical fitting result for liquid Fe 84 C 16 , compared with the velocity of liquid Fe (black curve) [8] . 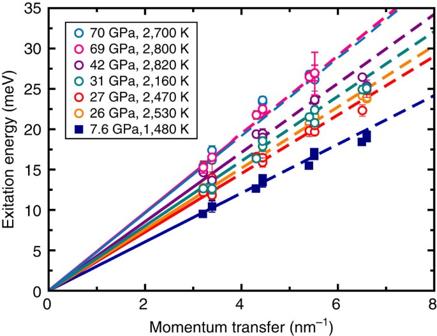Figure 4: Longitudinal acoustic phonon dispersion of liquid Fe84C16. The dispersion data were obtained at pressures from 7.6 to 70 GPa. Only data collected with the low momentum transfer (<3.5 nm−1) were used to determine the velocity to avoid possible anomalous dispersion for liquid (see Methods). Full size image Figure 4: Longitudinal acoustic phonon dispersion of liquid Fe 84 C 16 . The dispersion data were obtained at pressures from 7.6 to 70 GPa. Only data collected with the low momentum transfer (<3.5 nm −1 ) were used to determine the velocity to avoid possible anomalous dispersion for liquid (see Methods). 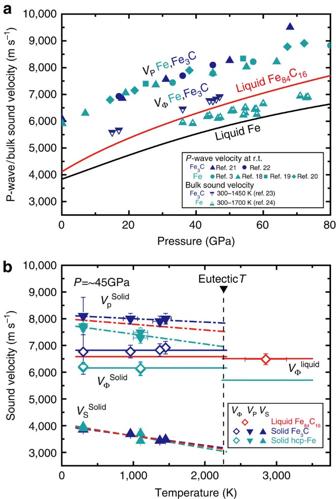Figure 5: Comparison of velocities between liquid and solid Fe–C alloys. (a), P-wave velocities (VP) and bulk sound velocities (VΦ) of solid Fe (turquoise)3,18,19,20,24and Fe3C (blue)21,22,23were determined by previous IXS and nuclear inelastic scattering (NIS) measurements. TheVPfor liquid Fe is from shock-wave study8. (b), Temperature effects on the sound velocities of Fe–C alloys at∼45 GPa. TheVP(=VΦ) of liquid Fe84C16and liquid Fe is from the present work at 42 GPa and shock-wave data8, respectively. TheVP, shear velocity (VS), andVΦfor solid Fe and Fe3C were reported by NIS measurements23,24. Red lines for fictional solid Fe84C16are estimated from a linear relationship between Fe and Fe3C. Full size image Figure 5: Comparison of velocities between liquid and solid Fe–C alloys. ( a ), P-wave velocities ( V P ) and bulk sound velocities ( V Φ ) of solid Fe (turquoise) [3] , [18] , [19] , [20] , [24] and Fe 3 C (blue) [21] , [22] , [23] were determined by previous IXS and nuclear inelastic scattering (NIS) measurements. The V P for liquid Fe is from shock-wave study [8] . ( b ), Temperature effects on the sound velocities of Fe–C alloys at ∼ 45 GPa. The V P (= V Φ ) of liquid Fe 84 C 16 and liquid Fe is from the present work at 42 GPa and shock-wave data [8] , respectively. The V P , shear velocity ( V S ), and V Φ for solid Fe and Fe 3 C were reported by NIS measurements [23] , [24] . Red lines for fictional solid Fe 84 C 16 are estimated from a linear relationship between Fe and Fe 3 C. Full size image Earlier ultrasonic measurements performed below 10 GPa reported a change in V P by <2–3% per 1,000 K for liquid Fe–S alloys [4] , [5] . Theoretical calculations [25] , [26] , [27] and shock compression data [8] on liquid Fe and Fe–S alloy demonstrated even smaller effects above 100 GPa (<0.5% by 1,000 K). It is therefore very likely that the V P of liquid Fe 84 C 16 is also not sensitive to temperature with the temperature effect much smaller than the uncertainty in the present velocity determinations (±3%). Thermodynamical equation of state V P of a liquid can be described using the Murnaghan equation of state [4] (Methods) as; where K S and K′ S are adiabatic bulk modulus and its pressure derivative, respectively (zero subscripts denote values at 1 bar and T = T 0 ). Here, consistent with the discussion above, we neglect the temperature dependence of our V P data, while ρ 0 is taken to be temperature dependent [16] (Methods). We fit equation (1) to our P – V P data for liquid Fe 84 C 16 and find K S0 =110±9 GPa and K ′ S =5.14±0.30 when T 0 =2,500 K ( Supplementary Table 2 and Supplementary Fig. 2 ). The choice of T 0 and, accordingly, the variation in ρ 0 practically changed K S0 and K ′ S0 as (∂ K S0 /∂ T )=−9.4 × 10 −3 GPa K −1 and (∂ K ′ S0 /∂ T ) =−2.7 × 10 −4 K −1 . Our value for K S0 is similar to that for liquid iron [8] but for K ′ S is higher than that for pure iron, K ′ S =4.7. This suggests that liquid Fe 84 C 16 becomes progressively stiffer than liquid Fe with increasing pressure. We also found V P0 =4,121±177 m s −1 for liquid Fe 84 C 16 from K S0 and ρ 0 , in good agreement with a previous study [28] of liquid Fe 86 C 14 at 1 bar (4,050 m s −1 ) and faster than V P0 =3,860 m s −1 for liquid Fe (ref. 8 ). To compare the present results with earlier density measurements of liquid Fe–C alloys at high pressure [29] , [30] the isothermal bulk modulus for liquid Fe 84 C 16 is estimated to be K T0 =100 (82) GPa at 1,500 K (2,500 K) from our determination of K S combined with Grüneisen parameter γ 0 =1.74 (ref. 8 ) and thermal expansion coefficient [16] (Methods). When applying C P / C V =1.125 at 1,820 K for liquid Fe 86 C 14 derived from theoretical calculations [31] , K T0 =106–98 GPa is obtained at the same temperature range. These K T0 values for liquid Fe 84 C 16 are similar to K T0 =95–63 GPa for liquid Fe at 1,500–2,500 K (ref. 8 ) On the other hand, they are significantly larger than K T0 =55.4 GPa for liquid Fe 86 C 14 at 1,500 K and K T0 =50 GPa for liquid Fe 75 C 25 at 1,973 K from previous density measurements [29] , [30] . However, the calculated density for Fe 84 C 16 using the present EoS are in reasonable agreement with the previous density measurements of Fe 75 C 25 (ref. 29 ) ( Fig. 6 ). The disagreement of elastic parameters with such earlier experiments may be attributed either to the limited pressure range of the previous density determinations, or to a different structure or magnetic (or electronic) change in the state of the liquid Fe–C at low pressure, as has been suggested from the change in compressional behaviour of liquid Fe 78 C 22 around 5 GPa (ref. 6 ). Our data were collected above 7.6 GPa, so that the physical properties of liquid Fe–C obtained here should be more applicable to the Earth’s core. 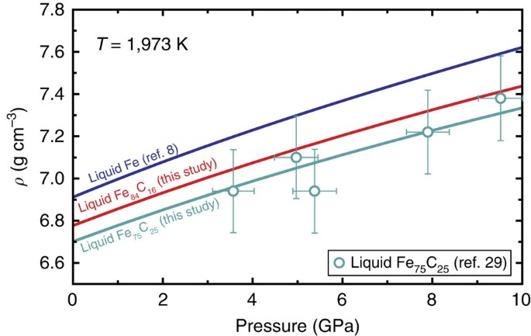Figure 6: Comparison with previous density measurements. Blue and red curves demonstrate calculated densities at 1,973 K for liquid Fe (ref.8) and Fe84C16(present study). The density of liquid Fe75C25(turquoise curve) is estimated assuming linear compositional dependence between pure Fe and Fe75C25, which shows good agreement with the previous measurements at 1,973 K (ref.29). Figure 6: Comparison with previous density measurements. Blue and red curves demonstrate calculated densities at 1,973 K for liquid Fe (ref. 8 ) and Fe 84 C 16 (present study). The density of liquid Fe 75 C 25 (turquoise curve) is estimated assuming linear compositional dependence between pure Fe and Fe 75 C 25 , which shows good agreement with the previous measurements at 1,973 K (ref. 29 ). Full size image ρ of liquid Fe 84 C 16 is then given, using the elastic parameters determined above, by; Equations (1) and (2) give the V P and ρ profiles for adiabatic compression (Methods), assuming γ 0 =1.74, the same as that of liquid Fe (ref. 8 ) ( Fig. 7 ). We find V P =9,200 m s −1 and ρ =9.82–9.61 g cm −3 at the core-mantle boundary (CMB) for T CMB =3,600–4,300 K (refs 32 , 33 ) This indicates that V P of liquid Fe 84 C 16 is 19.6% faster than that of liquid Fe at the CMB [8] , implying that the addition of 1 at.% carbon increases the V P of liquid Fe by 1.2%. The extrapolation of the present experimental data using the Murnaghan equation of state may overestimate the V P by 2−4% at the CMB ( Supplementary Note 1 and Supplementary Fig. 3 ), but, even if this is the case, 1 at.% carbon enhances the V P of liquid Fe by as large as 0.8%. Indeed, the effect of carbon is much larger than a recent theoretical prediction of only 0.2% increase in velocity per 1 at.% carbon at 136 GPa (ref. 34 ). On the other hand, our data show that the incorporation of 1 at.% carbon reduces the density of liquid Fe by 0.6–0.7%, while theory suggested only 0.3% density reduction by 1 at.% carbon [34] . 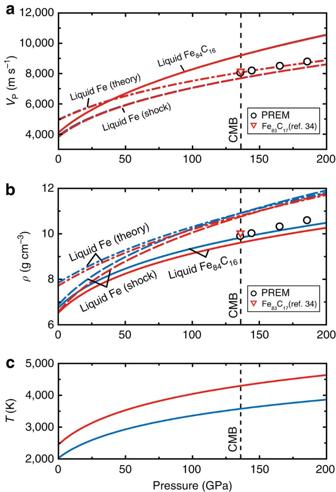Figure 7: Velocity and density of liquid Fe84C16extrapolated to core pressures. The P-wave velocity (a) and density (b) profiles of liquid Fe84C16are calculated along two adiabatic temperature curves (c) of 3,600 K (blue) and 4,300 K (red) at the CMB. Those for liquid Fe are from shock-compression experiments8and theoretical calculations26. The velocity and density for liquid Fe83C17at the CMB (4,300 K) are by theory34. PREM denotes seismologically deduced Preliminary Reference Earth model35. Figure 7: Velocity and density of liquid Fe 84 C 16 extrapolated to core pressures. The P-wave velocity ( a ) and density ( b ) profiles of liquid Fe 84 C 16 are calculated along two adiabatic temperature curves ( c ) of 3,600 K (blue) and 4,300 K (red) at the CMB. Those for liquid Fe are from shock-compression experiments [8] and theoretical calculations [26] . The velocity and density for liquid Fe 83 C 17 at the CMB (4,300 K) are by theory [34] . PREM denotes seismologically deduced Preliminary Reference Earth model [35] . Full size image We now compare the sound velocity and density of liquid Fe 84 C 16 and liquid Fe with the seismologically based PREM model [35] for the outer core ( Fig. 8 ). The V P and ρ of liquid Fe are 4.6% slower and 10.1–8.6% denser, respectively, than the PREM at the CMB (3,600–4,300 K). To match the PREM values, considering the uncertainty of data extrapolation to higher pressures ( Supplementary Note 1 ), only 5.2–4.0 at.% (1.2–0.9 wt.%) carbon is required to match the velocity, whereas 15.4–12.0 at.% (3.8–2.9 wt.%) carbon is necessary to account for the density. Therefore, carbon cannot be a predominant light element in the outer core. 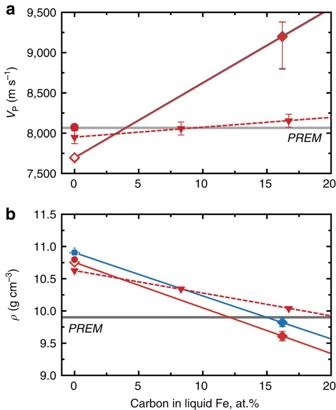Figure 8: Effect of carbon on the velocity and density of liquid Fe at 136 GPa. (a) Velocity and (b) density for liquid Fe84C16atTCMB=4,300 K (red) and 3,600 K (blue). Present results (closed diamonds, solid curves) are compared with theoretical calculations34(triangles, broken curve). The data for pure Fe are from shock compression study8(open diamonds) and theoretical calculations26(closed circles). PREM denotes seismological observations35at the CMB. Figure 8: Effect of carbon on the velocity and density of liquid Fe at 136 GPa. ( a ) Velocity and ( b ) density for liquid Fe 84 C 16 at T CMB =4,300 K (red) and 3,600 K (blue). Present results (closed diamonds, solid curves) are compared with theoretical calculations [34] (triangles, broken curve). The data for pure Fe are from shock compression study [8] (open diamonds) and theoretical calculations [26] (closed circles). PREM denotes seismological observations [35] at the CMB. Full size image These results suggest there is <5.2 at.% (1.2 wt.%) carbon in the outer core, consistent with the previous cosmochemical and geochemical arguments. In particular, the silicate portion of the Earth exhibits much higher 13 C/ 12 C isotopic ratio than that of Mars, Vesta and chondrite meteorites, as may be attributed to a strong enrichment of 12 C in core-forming metals [9] . The carbon isotopic fractionation that occurred during continuous core-formation process proposed previously [36] , [37] will give a reasonable 13 C/ 12 C ratio in the silicate Earth, and yields 1 wt.% carbon in the core [9] . In addition, Wood et al. [9] demonstrated that carbon strongly affects the chemical activity of Mo and W in liquid metal, so that their abundance in the mantle can be explained by partitioning between silicate melt and core-forming metal with ∼ 0.6 wt.% carbon. It has been repeatedly suggested that the inner core may be composed of Fe 7 C 3 , which accounts for high Poisson’s ratio observed [14] , [15] . The crystallization of solid Fe 7 C 3 from a liquid outer core with <1.2 wt.% carbon may still be possible if sulfur is also included in the core [38] . High P–T generation Molten Fe–C alloy was obtained at high P–T in an external-resistance-heated (EH) or laser-heated (LH) diamond-anvil cell (DAC; Supplementary Table 1 ) using facilities installed at SPring-8. A disc of pre-synthesized Fe 84 C 16 sample, 20–25 μm thick and 100–120 μm in diameter, was loaded into a hole of a rhenium gasket, together with two 12–17 μm thick single-crystal Al 2 O 3 sapphire discs that served as both thermal and chemical insulators. The sample was compressed with 300 μm culet diamond anvils to a pressure of interest before heating. In LH-DAC experiments, the sample was heated at high pressure from both sides by using two 100 W single-mode Yb fibre lasers (YLR-100-AC, IPG Photonics Corp.). The Gaussian-type energy distribution of the laser beam was converted into flat-top one with a refractive beam shaper (GBS-NIR-H3, Newport Corp.). A typical laser spot was 50–70 μm in diameter on the sample, much larger than X-ray beam size ( ∼ 17 μm). We determined temperature by a spetroradiometric method, and its variations within the area irradiated by X-rays and fluctuations during IXS measurements were <±10%. The pressure was obtained from the equation of state for Fe 3 C (ref. 39 ) from the lattice constant observed before melting at 1,800–2,500 K. Its error was derived from uncertainties in both temperature and the volume of Fe 3 C. A typical image of a sample recovered after the laser heating experiment at 70 GPa and 2,700 K is given in Supplementary Fig. 4 . Only run #FeC08 was conducted in an EH-DAC. The whole sample was homogeneously heated by a platinum-resistance heater placed around the diamonds. The temperature was obtained with a Pt-Rh (type-R) thermocouple whose junction was in contact with the diamond near a sample chamber. The temperature uncertainty was <20 K. We determined the pressure based on the Raman shift of a diamond anvil [40] before heating at 300 K, whose uncertainty may be as much as ±20%. IXS measurements The sound velocity of liquid Fe–C alloy was determined in the DAC by high-resolution IXS spectroscopy at the beamline BL35XU, SPring-8 (ref. 41 ). Both LH- and EH-DACs were placed into vacuum chambers to minimize background scattering by air. The measurements were carried out with ∼ 2.8 meV energy resolution using Si (999) backscattering geometry at 17.79 keV. The experimental energy resolutions were determined using scattering from Polymethyl–methacrylate. The incident X-ray beam was focused to about 17 μm size (full width at half maximum) in both horizontal and vertical directions by using Kirkpatrick–Baez mirrors [42] . The X-ray beam size was much smaller than heated area (50–70 μm for LH-DAC). Scattered photons were collected by an array of 12 spherical Si analyzers leading to 12 independent spectra at momentum transfers ( Q ) between 3.2 and 6.6 nm −1 with a resolution Δ Q ∼ 0.45 nm −1 (full width) that was set by slits in front of the analyzer array. The energy transfer range of ±30 (or −10 to ±30) meV was scanned for 1–3 h. Before and after IXS data collections, sample melting was confirmed by X-ray diffraction data ( Fig. 2 ) that was collected, in situ , by switching a detector to a flat panel area detector (C9732DK, Hamamatsu Photonics K.K.) [43] . The IXS spectra included three (sometimes five) peaks ( Fig. 1 ) of Stokes and anti-Stokes components of the longitudinal acoustic (LA) phonon mode from the sample (sometimes also from a diamond), and a quasi-elastic contribution near zero energy transfer. These spectra were fitted with the damped harmonic oscillator (DHO) mode [44] for acoustic phonon modes and with Lorenzian function for quasi-elastic peaks convolved by experimental resolution function. The DHO model function can be described as; where A Q , Γ Q , Ω Q , k B and ħ are the amplitude, width, and energy of inelastic modes, Boltzmann constant and Planck constant, respectively. In the fitting, temperature T was fixed at a sample temperature obtained by a spetroradiometric method or a thermocouple. The excitation energy modes appearing at both Stokes and anti-Stokes sides correspond to the phonon creation and annihilation, respectively. With increasing temperature, as given by the Bose function in equation (3), the intensities of such Stokes and anti-Stokes peaks become similar to each other. A symmetric shape of the present IXS spectra therefore assures that the IXS signals originated from a high-temperature area. The peak at a finite energy transfer gives the frequency of each mode ( Fig. 1 ). The excitation energies for the LA phonon mode of liquid Fe 84 C 16 obtained in a pressure range of 7.6–70 GPa are plotted as a function of momentum transfer ( Q ) in Fig. 4 . The compressional sound wave or P-wave velocity ( V P ) corresponds to the long-wavelength LA velocity at Q →0 limits; We made a linear fit to the data obtained at low Q below 3.5 nm −1 to determine the P-wave velocity ( Supplementary Table 1 ), because positive dispersion can appear at higher Q >>3 nm −1 (ref. 45 ). For comparison, the results based on a sine-curve fit to all Q -range data, as is usually applied for polycrystalline samples in similar high-pressure IXS measurements [46] , are also given in Supplementary Table 1 . In general, the error bars of the two determinations of V P overlap, though the sine fit to large Q does give slightly larger V P , as would qualitatively be expected from previous measurements on liquid iron [47] . Equation of state for liquid Fe 84 C 16 We constructed an equation of state (EoS) for liquid Fe 84 C 16 to extrapolate the present V P data and to estimate its density at the core pressure range. V P of liquid can be written as; The pressure dependence of K S is assumed to be where K′ S is the pressure derivative of K S and pressure and subscript zero indicates a value at 1 bar. The adiabatic Murnaghan EoS can be described as (for example, ref. 4 ); Equation (5) is thus rewritten as; The temperature effect on ρ 0 can be expressed by; The thermal expansion coefficient α is also dependent on temperature as; where a and b are constants. Previous density measurements [16] of liquid Fe–C alloys at 1 bar give a =6.424 × 10 −5 K −1 and b =0.606 × 10 −8 K −2 for liquid Fe 84 C 16 using ρ 0 =6.505 g cm −3 at T 0 =2,500 K as a reference. The result of fitting equation (8) to the present P − V P data is given in Fig. 3 . Isothermal bulk modulus We estimate isothermal bulk modulus K T from isentropic bulk modulus K S in two ways. The relationship between these two is described as follows; where C P and C V are heat capacities at constant pressure and volume, respectively. Although γ for liquid Fe–C alloys is not known, γ 0 =1.74 has been reported for liquid Fe at 1 bar and 1,811 K (ref. 8 ) It is close to 1.58 for liquid Fe 90 O 8 S 2 estimated from the shock compression data set [48] . Extrapolation of present data to core pressures With the EoSs determined above (equations (7) and (8)), we extrapolate the P-wave velocity and density of liquid Fe 84 C 16 to the core pressure range along adiabatic compression, in which temperature is given by; Assuming γ = γ 0 × ( ρ 0 / ρ ), temperature is simply represented as; γ 0 is fixed at 1.74 previously obtained for liquid Fe (ref. 8 ). Using the temperature dependence of K S0 and ρ 0 shown above, we calculate density, velocity and temperature profiles along adiabatic compression with various reference temperatures at the CMB. The adiabatic compression profiles of liquid Fe 84 C 16 for the low ( T 0 =2,045 K and T CMB =3,600 K) [32] and high ( T 0 =2,457 K and T CMB =4,300 K) [33] temperature cases are calculated in Fig. 7 . How to cite this article: Nakajima, Y. et al. Carbon-depleted outer core revealed by sound velocity measurements of liquid iron–carbon alloy. Nat. Commun. 6:8942 doi: 10.1038/ncomms9942 (2015).